Brown fat in a protoendothermic mammal fuels eutherian evolution Endothermy has facilitated mammalian species radiation, but the sequence of events leading to sustained thermogenesis is debated in multiple evolutionary models. Here we study the Lesser hedgehog tenrec ( Echinops telfairi ), a phylogenetically ancient, ‘protoendothermic’ eutherian mammal, in which constantly high body temperatures are reported only during reproduction. Evidence for nonshivering thermogenesis is found in vivo during periodic ectothermic–endothermic transitions. Anatomical studies reveal large brown fat-like structures in the proximity of the reproductive organs, suggesting physiological significance for parental care. Biochemical analysis demonstrates high mitochondrial proton leak catalysed by an uncoupling protein 1 ortholog. Strikingly, bioenergetic profiling of tenrec uncoupling protein 1 reveals similar thermogenic potency as modern mouse uncoupling protein 1, despite the large phylogenetic distance. The discovery of functional brown adipose tissue in this ‘protoendothermic’ mammal links nonshivering thermogenesis directly to the roots of eutherian evolution, suggesting physiological importance prior to sustained body temperatures and migration to the cold. The discovery of evolutionary events that allowed mammals to generate and sustain high body temperatures (Tbs) is one of the most intriguing, and still unresolved, questions in the evolutionary physiology of vertebrates [1] , [2] , [3] . A variety of evolutionary models promote high Tb as a facilitator of higher resting metabolic rate (RMR), which may represent selection benefits [4] , [5] , [6] . Other models, however, favour the idea that high metabolic rates (MRs) are instead a consequence of increased exercise, increased brain size and high aerobic capacity, arguing that the advantages of high Tb per se are insufficient to compensate for the energetic costs [7] . Evolutionary ecologists agree that decreasing juvenile mortality and accelerating growth to maturity are among the most effective ways of increasing species fitness [8] , leading to the hypothesis that the benefits of parental care are key in the understanding of endothermic convergence between mammals and birds [2] , [5] . There is an increasing palaeontological evidence that early mammals were rather small, and, though not having to cope with extreme cold climates, the evolution of homoeothermic endothermy at unfavourable body surface-to-volume ratios likely involved enhanced insulation, and improved thermoregulatory abilities [6] . Recent eutherian mammals use an array of behavioural, vasomotory and thermogenic processes, including both shivering and nonshivering thermogenesis (NST) (ref. 9 ), to maintain high Tbs in the cold. In many small-sized eutherian species, the major source of NST is brown adipose tissue (BAT) (ref. 10 ), which is characterized by high mitochondrial content and the expression of uncoupling protein 1 (UCP1) (ref. 11 ). UCP1 transports protons directly across the mitochondrial inner membrane, bypassing ATP production, thereby dissipating proton motive force as heat. For small-sized mammalian species, the significance of BAT for the maintenance of high Tbs in the cold and for the arousal from torpid or hibernating states is well established [9] , [12] . Yet an ultimate cause favouring the evolution of distinct anatomical depots with specific thermogenic properties has yet to be revealed. This is particularly intriguing as the evolutionary history of UCP1 dates back to the origin of teleost fishes about 420 million years ago [13] . To gain insight into the origins of NST and its role in the evolution of eutherian homoeothermic endothermy, we study the Lesser hedgehog tenrec, Echinops telfairi , a member of the phylogenetically ancient afrotherian clade of eutherian mammals. The tenrec is considered ‘protoendothermic’ as Tb tracks closely to ambient temperature (Ta) in reptilian-like patterns, with only a few hours per day of endothermic periods [14] . Despite seemingly primitive thermogenic competence, however, tenrec females maintain constantly high Tbs (~33 °C) during pregnancy and periods of parental care [15] . Here we describe the unexpected identification of potent BAT in the Lesser hedgehog tenrec ( E. telfairi ) and its role in temperature regulation. Bioenergtic profiling of tenrec BAT and UCP1 reveals activities that are similar to those of modern eutherian mammals such as mouse ( Mus musculus ). Thermoregulation in E. telfairi Similar to observations in the wild [14] , all tenrecs in captivity were colder than 30 °C for most of the time, irrespective of Ta ( Fig. 1a–c ). Tb nadirs decreased in the cold and were paralleled by a corresponding expansion of daily Tb amplitudes ( Fig. 1b–f ). On average, minimal Tb was always 0.4–1.6 °C higher than Ta. Tb maximized at 32 °C, irrespective of Ta, reflecting the lowest Tbs of eutherians among egg-laying monotremes and ‘poikilothermic’ naked mole rats ( Heterocephalus glaber ) [16] . The brief daily episodes of high Tb were regularly observed during the dark phase of the light/dark cycle, but tenrecs never remained homoeothermic at this level for more than 6 h. Notably, all tenrecs were capable of rewarming from hypothermia in the absence of exogenous sources of heat. We frequently observed animals feeding while still at low Tb, and then rewarming to >30 °C, which was always accompanied by visible shivering. 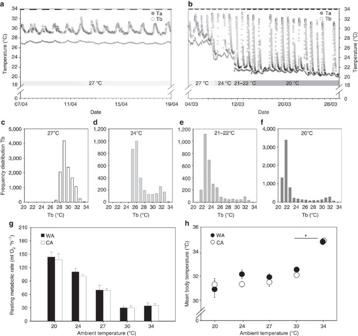Figure 1: Thermoregulation inE. telfairi. (a,b) Representative Tb traces of a WA (a, Ta =27 °C) and a successively CA (b, 27 °C to 20 °C) tenrec. (c–f) Tb histograms at different Tas (N=6 animals per chart). (g,h) Mean RMR (g) and Tb (h) over a range of Tas, determining the TNZ (WA:N=5–6; CA:N=6; *P=0.001, Student’st-test, data represent means±s.e.m.). Figure 1: Thermoregulation in E. telfairi . ( a , b ) Representative Tb traces of a WA ( a , Ta =27 °C) and a successively CA ( b , 27 °C to 20 °C) tenrec. ( c – f ) Tb histograms at different Tas ( N =6 animals per chart). ( g , h ) Mean RMR ( g ) and Tb ( h ) over a range of Tas, determining the TNZ (WA: N =5–6; CA: N =6; * P =0.001, Student’s t -test, data represent means±s.e.m.). Full size image Using combined indirect calorimetry and Tb telemetry, the thermoneutral zone (TNZ) of warm (WA) and cold acclimated (CA) E. telfairi was determined for the first time, revealing a thermal window of 30 to <34 °C in both groups ( Fig. 1g ). The RMRs at thermoneutrality were exceptionally low as compared with similar sized members of higher mammalian orders [17] . Below 30 °C, cold-induced regulatory thermogenesis was evident by an increase in RMRs with decreasing Ta. In contrast, at 34 °C, cessation of active thermoregulation was evident by a diminished Tb–Ta gradient ( Fig. 1h ), with animals obviously suffering from heat stress. In vivo evidence for NST in E. telfairi The heat production patterns of E. telfairi were recorded for at least two episodes of arousal from hypometabolism for each individual ( Fig. 2a ). The minimal MR before arousal was about 9 ml O 2 h −1 (~50 mW), equivalent to an almost 10-fold reduction compared with resting heat production levels for each group ( Fig. 2b ). 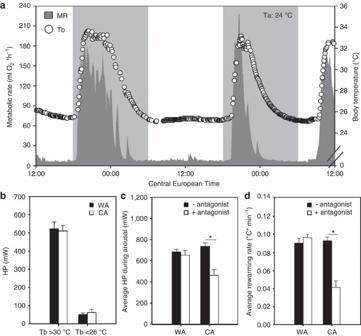Figure 2: Heat production (HP) during episodic rewarming. (a) Temporal-resolved thermogenic profile, including heating events from hypothermia (shaded area: lights off). (b) Resting HP during euthermia and hypometabolism. (c,d) Average HP and average rewarming rates during arousal, calculated over the same temperature range of 25.5–29.75 °C, with or without injection of the β3-adrenergic antagonist SR 59230A (N=5 per group; *P<0.05, pairedt-test, data represent means±s.e.m.). Figure 2: Heat production (HP) during episodic rewarming. ( a ) Temporal-resolved thermogenic profile, including heating events from hypothermia (shaded area: lights off). ( b ) Resting HP during euthermia and hypometabolism. ( c , d ) Average HP and average rewarming rates during arousal, calculated over the same temperature range of 25.5–29.75 °C, with or without injection of the β3-adrenergic antagonist SR 59230A ( N =5 per group; * P <0.05, paired t -test, data represent means±s.e.m.). Full size image In modern eutherian mammals, classical NST is mediated via β3-adrenergic receptor signalling in BAT (ref. 9 ). In CA tenrecs, treatment with the β3-adrenergic antagonist SR 59230A at the onset of arousal from hypometabolism significantly reduced heat production ( Fig. 2c , P <0.05, paired t -test) and rewarming rates ( Fig. 2d , P <0.05, paired t -test), supporting inhibition of adaptive NST that classically replaces shivering thermogenesis in the cold. Identification of functional BAT Post-mortem anatomical inspection identified typical small brown fat patches in the dorso-cervical and axillar region, whereas, surprisingly, a large depot of brown fat-like tissue was located in the abdominal region, adjacent to the reproductive organs (~60–70% of total BAT, Fig. 3a ). The presence of β3-adrenoreceptors was corroborated by immunological detection in brown fat homogenates. Although β3-adrenoreceptor protein content was unchanged in response to cold acclimation ( Fig. 3b ), differential recruitment of NST was reflected in increased oxidative capacity of BAT tissue and BAT mitochondria of CA tenrecs (measured as cytochrome- c oxidase (COX) activity, Fig. 3e–g ). Further immunological analysis of this tissue suggested cold-induced expression of UCP1 ( Fig. 3c ), and this detection was confirmed using an anti-hamster UCP1 antibody and by cloning the tenrec UCP1 cDNA. 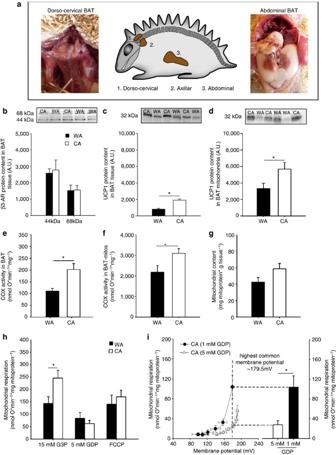Figure 3: Morphological and molecular and biochemical evidence for functional BAT. (a) Anatomical location of tenrec BAT. (b–d) Immunological detection of (b) β3-adrenoreceptor protein subunits in tissue homogenates, (c) UCP1 in tissue homogenates and (d) in isolated mitochondria, revealing cold induction. (e,f) COX activity in BAT homogenates and isolated mitochondria, demonstrating increased oxidative capacity in the cold. (g) Mitochondrial content, estimated from the ratio of tissue to mitochondrial COX activity. (*P<0.05, Student’st-test). (h,i) Mitochondria respiration rates (N=4–5, *P<0.05, Student’st-test) and proton leak kinetics of isolated BAT mitochondria in response to GDP, FCCP and 5 mM GDP (N=4–5, *P<0.05, pairedt-test, data represent means±s.e.m.). Figure 3: Morphological and molecular and biochemical evidence for functional BAT. ( a ) Anatomical location of tenrec BAT. ( b – d ) Immunological detection of ( b ) β3-adrenoreceptor protein subunits in tissue homogenates, ( c ) UCP1 in tissue homogenates and ( d ) in isolated mitochondria, revealing cold induction. ( e , f ) COX activity in BAT homogenates and isolated mitochondria, demonstrating increased oxidative capacity in the cold. ( g ) Mitochondrial content, estimated from the ratio of tissue to mitochondrial COX activity. (* P <0.05, Student’s t -test). ( h , i ) Mitochondria respiration rates ( N =4–5, * P <0.05, Student’s t -test) and proton leak kinetics of isolated BAT mitochondria in response to GDP, FCCP and 5 mM GDP ( N =4–5, * P <0.05, paired t -test, data represent means±s.e.m.). Full size image Intact BAT mitochondria, energized with glycerol-3-phosphate in a temperature-controlled chamber at 32 °C, showed significantly higher respiration rates in CA tenrecs ( Fig. 3h ). This difference was most likely caused by UCP1 proton leak activity as addition of guanosine diphosphate (GDP), an UCP1 inhibitor, decreased the respiration rate by 40% and 76% in WA and CA animals, respectively. Next, we assessed mitochondrial proton conductance by measuring proton leak kinetics as flux-force curves of mitochondrial respiration and membrane potential ( Fig. 3i ). As mitochondria were fully uncoupled under basal conditions, measurement of proton motive force (membrane potential in the presence of nigericin) required the addition of 1 mM GDP. Increasing the concentration to 5 mM GDP fully recoupled the mitochondria, shifting proton leak kinetics significantly downwards, demonstrating that UCP1 catalyses the major proportion of proton conductance. Bioenergetic characterization of tenrec UCP1 For further comparative bioenergetic characterization, tenrec UCP1 (etUCP1) and mouse UCP1 (mUCP1) orthologs were stably transfected in HEK293 cells and functionally analysed using plate-based respirometry of intact cells. Comparing the respiration profiles and coupling efficiencies of HEK293 cells in the presence and absence of BSA confirmed that residual fatty acids induced proton leak respiration (oligomycin-insensitive) selectively in UCP1-containing cells ( Fig. 4a ). Residual fatty acids in the absence of BSA, however, were also oxidized and contributed to mitochondrial substrate oxidation, as judged by increased FCCP-induced respiration ( Fig. 4a ). Specific activation of UCP1 was confirmed using the retinoic acid analogue TTNPB, which activates UCP1 but is not metabolized ( Fig. 4c ) [18] . Furthermore, we activated UCP1 in the intact cell with nonanoic acids that do not require conjugation to BSA and readily diffuse into the HEK293 cells. The bioenergetic profile of tenrec and mouse UCP1 revealed a similar dose dependency for these small molecular activators ( Fig. 4d ). Notably, there was no activator effect on wild-type HEK293 cells. As both of the UCP1 proteins have similar functional properties, BAT in the two distantly related species reflects an orthologous condition. 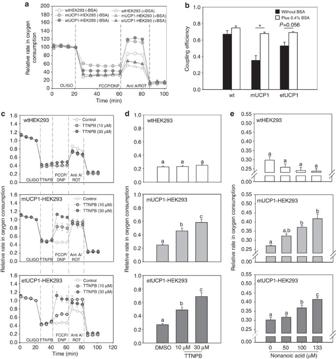Figure 4: Comparative bioenergetic profiling of tenrec and mouse UCP1 in HEK293 cells. (a) Representative traces of normalized plate-based respirometry, showing basal respiration, proton leak respiration (after oligomycin treatment), maximal substrate oxidation (FCCP or DNP) and non-mitochondrial respiration (antimycin A/rotenone). (b) BSA-sensitive coupling efficiency (white bars) of mouse UCP1 (mUCP1) and tenrec UCP1 (etUCP1)-containing HEK293 cells (N=5 per group and condition; *P<0.05, Student’st-test). (c–e) Specific activation of stably expressed mUCP1 and etUCP1, in comparison with wild-type HEK293 (wtHEK293) (N=5–6,P<0.001, one-way ANOVA, lowercase letters indicate statistical difference atP<0.005, data represent means±s.e.m.). Figure 4: Comparative bioenergetic profiling of tenrec and mouse UCP1 in HEK293 cells. ( a ) Representative traces of normalized plate-based respirometry, showing basal respiration, proton leak respiration (after oligomycin treatment), maximal substrate oxidation (FCCP or DNP) and non-mitochondrial respiration (antimycin A/rotenone). ( b ) BSA-sensitive coupling efficiency (white bars) of mouse UCP1 (mUCP1) and tenrec UCP1 (etUCP1)-containing HEK293 cells ( N =5 per group and condition; * P <0.05, Student’s t -test). ( c – e ) Specific activation of stably expressed mUCP1 and etUCP1, in comparison with wild-type HEK293 (wtHEK293) ( N =5–6, P <0.001, one-way ANOVA, lowercase letters indicate statistical difference at P <0.005, data represent means±s.e.m.). Full size image Comparative molecular characterization of tenrec versus mouse UCP1 Despite demonstrating similar molecular activators of etUCP1 and mUCP1, the question remained whether these orthologs differ in their specific activities as a result of their distant phylogenetic relationship. For comparative molecular characterization of etUCP1, we isolated mitochondria from HEK293 cells and measured proton leak kinetics of wild-type mouse and tenrec UCP1-containing HEK293 cell mitochondria ( Fig. 5a–c ). Basal, palmitate-induced and GDP-inhibited UCP1 activity was similar to that of native BAT mitochondria. The decrease of proton leak to wild-type levels by addition of GDP demonstrated full inhibition of both mUCP1 and etUCP1. For quantitative functional comparison of etUCP1 and mUCP1, we normalized the proton leak curves to UCP1 content using overexpressed and purified UCP1 orthologs as mass standards ( Supplementary Fig. S1 ). Next, we subtracted the GDP-insensitive basal proton leak from the UCP1 leak under control conditions. The resulting specific UCP1 catalytic activity did not differ between mouse and tenrec UCP1 ( Fig. 5d ), despite the large phylogenetic distance between the Afrotheria and the modern Eutheria. 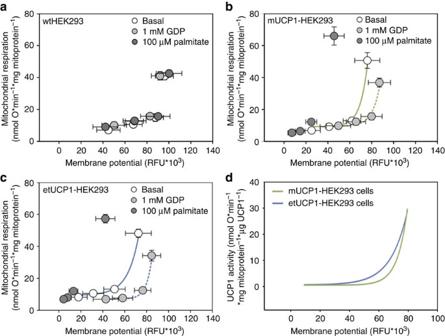Figure 5: Determination of catalytic centre activities of tenrec and mouse UCP1 in isolated HEK293 cell mitochondria. (a–c) Proton leak kinetics of wild-type (wt), mouse UCP1 (mUCP1) and tenrec UCP1 (etUCP1) HEK293 cells, under basal conditions after activation with 100 μM palmitate and after inhibition with 1 mM GDP (N=6 per group and condition) (d) Specific UCP1 activity curves reveal similar catalytic power of tenrec and mouse UCP1 (derived fromFig. 4b). Figure 5: Determination of catalytic centre activities of tenrec and mouse UCP1 in isolated HEK293 cell mitochondria. ( a – c ) Proton leak kinetics of wild-type (wt), mouse UCP1 (mUCP1) and tenrec UCP1 (etUCP1) HEK293 cells, under basal conditions after activation with 100 μM palmitate and after inhibition with 1 mM GDP ( N =6 per group and condition) ( d ) Specific UCP1 activity curves reveal similar catalytic power of tenrec and mouse UCP1 (derived from Fig. 4b ). Full size image Obligatory thermogenesis in mammals conveys energetic costs that need to be outweighed by fitness gain, a tenet that has provoked controversial discussions on the events leading to the evolution of sustained endothermy [1] , [2] , [3] , [4] , [5] , [6] , [7] , [8] . This study on the ‘protoendothermic’ tenrec posits good molecular arguments that potent BAT-derived thermogenesis pre-dated the appearance of systemic homoeothermic endothermy at the roots of eutherian evolution. Contrasting the traditional view that BAT-like thermogenic mechanisms evolved and improved secondary to sustained high MRs facilitating eutherian niche expansion, the opportunistic recruitment of thermogenesis, notably including BAT, may have been the driving force for sustained eutherian endothermy before migration to colder environments (as outlined in Fig. 6 ). 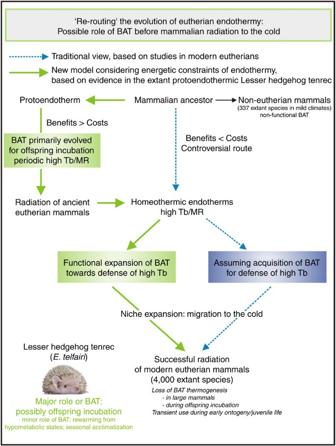Figure 6: A new model of thermogenic evolution in eutherian mammals. In this possible evolutionary scenario, potent BAT-derived thermogenesis pre-dated the appearance of systemic homoeothermic endothermy at the roots of eutherian evolution, before migration to the cold. The opportunistic recruitment of thermogenesis, notably including BAT, during periods of parental care, may have been the driving force for sustained eutherian endothermy. Figure 6: A new model of thermogenic evolution in eutherian mammals. In this possible evolutionary scenario, potent BAT-derived thermogenesis pre-dated the appearance of systemic homoeothermic endothermy at the roots of eutherian evolution, before migration to the cold. The opportunistic recruitment of thermogenesis, notably including BAT, during periods of parental care, may have been the driving force for sustained eutherian endothermy. Full size image Although periodic endothermy of the tenrec is facilitated by BAT during intermittent episodes of homoeothermy, as shown in this study, prolonged endothermic episodes have only been reported during reproduction [15] . As judged from the anatomical distribution, BAT thermogenesis may be particularly relevant during periods of gamete and offspring incubation, and although impossible to prove, evolutionary selection may have favoured BAT NST for/by parental care. In modern eutheria, physiological expansion of BAT for maintenance of high Tb in the cold allowed global species radiation [9] , which appears more successful as compared with that of non-eutherian mammals possessing no functional BAT (as outlined in Fig. 6 ). Study animals and maintenance Experiments were performed on laboratory bred, adult Lesser hedgehog tenrecs ( E. telfairi ; N =8 females and 4 males) during their annual activity period. A detailed description of tenrec husbandry can be found in the Supplementary Methods . All animal experimental procedures were approved by the German Animal Welfare Authorities. Body-temperature recording Tenrecs were surgically implanted with temperature-sensitive transmitters (Model X; Mini Mitter, Sunriver, OR, USA; accuracy 0.1 °C) for monitoring abdominal core Tb. The surgery procedure and recovery phase are described in detail in the Supplementary Methods . Hereafter, six animals were randomly selected for the CA group ( N =5 females and 1 male) and stepwise acclimated to 20 °C (4 days at 24 °C, 3 days at 21–22 °C). The other six animals remained at 27 °C (WA group; N =3 females and 3 males). The average body mass of the animals was 133.3±29.1 g for the WA group (93.4–166.4 g) and 162.5±27.1 g (122.8–196.5 g) for the CA group ( P =0.102, Student’s t -test) and remained constant throughout the entire study. During long-term Tb recordings, Tb readings were obtained every 6 min for 7–12 days at a Ta of 27 °C, 3–4 days at 24 °C, 2–3 days at 21–22 °C and 3–6 days at 20 °C (only CA group). Resting metabolic rates MR measurements were based on the principle of indirect calorimetry using a two-channel, open-circuit respirometry system [19] . Tenrecs were transferred to metabolic cages (~5.0 l) equipped with bedding material and were placed inside a climate chamber. Air was drawn from the cages at a flow rate of 42 l h −1 chosen to maintain <1% oxygen depletion between the incurrent and excurrent air. On each measurement day, tenrecs were exposed for 4–5 h to only one of the following temperatures: 34, 30, 27, 24 and 20 °C, in random order. In between each measurement, tenrecs were allowed to recover for at least 2 days in their home cage. On each occasion, readings of MR (VO 2 consumption) and Tb were taken at 3–5-min intervals. Arousal and rewarming Animals became hypometabolic and hypothermic in the trials conducted at Tas <30 °C, and introduction of food to the cage was used to induce arousal. Following arousal, we obtained stable metabolic readings of resting animals at high Tbs (RMR, not post-absorptive). The comparison of induced versus spontaneous arousal and rewarming rates did not reveal group differences ( Supplementary Fig. S2 ). For pharmacological manipulation of BAT-derived NST, each tenrec received a single subcutaneous injection of the β3-adrenergic antagonist SR 59230A (3-(2-ethylphenoxy)-1-[[(1S)-1,2,3,4-tetrahydronaphth-1-yl]amino]-(2S)-2-propanol oxalate salt; Sigma) [20] at a dosage of 1 mg kg −1 . A detailed protocol is described in the Supplementary Methods . Presence of BAT and expression of UCP1 We dissected animals to identify and locate BAT depots. Tissue samples were collected and used to confirm the expression of UCP1 mRNA and protein. In brief, UCP1 cDNA was amplified using a reverse transcriptase (Super Script III First Strand cDNA Synthesis Super Mix for quantitative reverse transcriptase PCR; Invitrogen) and tenrec UCP1-specific primers (forward: 5′-GACTATGGGGGTGAAGATCTTC-3′; reverse: 5′-AAAGGCCGGCAGCCCTTCCTTG-3′), followed by a PCR using the same primer pair and a gel electrophoresis to validate UCP1 expression (GenBank: KC158558.1). The presence or absence of UCP1 protein was confirmed post mortem by immunological detection in BAT homogenate and BAT mitochondria. The membranes were probed with a rabbit anti-UCP1 polyclonal antibody (1:10,000; 3046; Chemicon), followed by the relevant fluorescence-conjugated secondary antibody. The expression of the β3-adrenergic receptor was confirmed using a goat polyclonal β3-adrenoreceptor primary antibody (1:200; Santa Cruz Biotechnology). COX activity and mitochondria isolation and respiration COX activity and mitochondrial respiration was measured polarographically [21] using a Clark-type oxygen electrode (Rank Brothers Ltd.) maintained at 25 °C (COX measurements) or 32 °C (mitochondrial respiration) as described in Supplementary Methods . BAT depots were removed (dorso-cervical, axillar and abdominal) and immediately placed in ice-cold isolation medium. Mitochondria were prepared by homogenization and differential centrifugation [22] . Proton leak kinetics The kinetics of mitochondrial proton leak were measured by determining the respiration rate required to drive the proton leak. Measurements were performed with 0.5 mg ml −1 BAT mitochondria in buffer containing 2 μM oligomycin, 100 nM nigericin (dissipating the pH gradient; Cadenas and Brand [23] ), 4.8 μM rotenone (inhibiting complex I) and 2.5 μM carboxyatractylate (inhibiting the adenine nucleotide translocase). The mitochondrial membrane potential was measured simultaneously by using an electrode sensitive to the potential-sensitive probe, triphenylmethylphosphonium (TPMP+). The TPMP+-sensitive electrode was calibrated with sequential additions of TPMP+ up to 2.5 μM, and succinate (4 mM) was added to initiate mitochondrial oxidation. Membrane potential and respiration were progressively inhibited through successive steady states with malonate up to 5 mM. Finally FCCP (0.3 μM) was added to dissipate the membrane potential and release TPMP+ from the mitochondria, allowing for correction of baseline drift. Respiration at each steady state was plotted against the corresponding membrane potential to determine the dependence of proton leak rate on the membrane potential. UCP1-dependent proton leak was determined in the presence of 1–5 mM GDP. Stable expression of etUCP1 in mammalian HEK293 cells For analysis of UCP1 in HEK293 cells, the tenrec UCP1 cds (GenBank: KC158558.1) was transcribed to cDNA, cloned into a pcDNA3 vector (Invitrogen; containing neomycin/geneticin-resistant genes), amplified, transfected into human embryo kidney cells (HEK293) and selected for stable expression [24] (culturing conditions can be found in the Supplementary Methods ). Seahorse experiments HEK293 cells were seeded as described in the Supplementary Methods . The XF24 plate was then transferred to a temperature-controlled (37 °C) XF24 Extracellular Flux analyser (Seahorse Bioscience), equilibrated for 10 min. Four assay cycles (1-min mix, 2-min wait and 3-min measuring period) were used to determine basal respiration, and then oligomycin (4 μM; inhibiting ATP synthase) was added by automatic pneumatic injection (three assay cycles). Next, different concentrations of TTNPB (4-[(E)-2-(5,6,7,8-tetrahydro-5,5,8,8-tetramethyl-2-naphthalenyl)-1-propenyl]benzoic acid) (0, 15 and 30 μM diluted in dimethylsulphoxide) or nonanoic acid (30, 50, 100 and 133 μM) were injected, followed by an injection of FCCP (carbonyl cyanide p-trifluoromethoxyphenylhydrazone) (0.5 μM) or DNP (2,4-dinitrophenol) (100 μM) to completely uncouple mitochondria. Each experimental trace was ended by final injection of a cocktail of rotenone (4 μM) and antimycin A (2 μM) to correct for non-mitochondrial respiratory rate. Coupling efficiency was calculated as the oligomycin-sensitive fraction of glucose/pyruvate-stimulated mitochondrial respiratory activity. Proton leak kinetics of isolated HEK293 cell mitochondria HEK293 cells were grown in bulk for isolation of mitochondria as described in the Supplementary Methods . Mitochondrial respiration and membrane potential were measured in KHE buffer (120 mM KCl, 5 mM KH 2 PO 4 , 3 mM HEPES, 1 mM EGTA and 0.3% BSA (w/v); pH 7.2 at room temperature) at a protein concentration of 0.8 mg ml −1 . The dye safranin O was used for the measurement of mitochondrial membrane potential. Safranin O changes fluorescence in a manner linearly proportional to the mitochondrial membrane potential [25] . The excitation and emission wavelengths were set to 533 and 576 nm, respectively, and measurements were performed in a 96-well plate at a gain of 500 and a focal height of 7.1 nm in a high-throughput-screening microplate reader (Pherastar FS; BMG Labtech). A total of 40 μg of mitochondrial protein was measured in 200 μl of KHE in the presence of 5 μM Safranin O, 4 μM rotenone, 1 μg μl −1 oligomycin and 100 nM nigericin, and GDP (1 mM) and palmitate (100 μm) were added when indicated. After incubation time, succinate (5 mM) was added to energize mitochondria. The induced membrane potential and respiration were subsequently inhibited by 2 mM titration steps of malonate (up to 6 mM). At the end of each run, the membrane potential was dissipated by addition of 0.3 μM FCCP. The relative changes in fluorescent signal are proportional to the membrane potential; larger changes in relative fluorescence units indicating higher membrane potentials after mitochondria energetization. Comparison of the safranin O signal before energetization and after dissipation of the membrane potential with FCCP allowed correction for drifts in the baseline fluorescent signal. In addition, background wells without mitochondria were measured for each condition to correct for fluorescence quenching effects. Recombinant UCP1 standard Construction of the UCP1 vector is described in the Supplementary Methods . Mouse UCP1 and tenrec UCP1 were expressed in Escherichia coli (strain C41 (DE3)), and inclusion bodies were isolated [26] , quantified and the purity determined (see Supplementary Fig. S1 and Supplementary Methods ). Statistical analysis The paired t -test was used to test for effects of the β3-adrenergic antagonist and GDP on proton leak curves within the CA and WA group, the Student’s t -tests were used to test for differences between the acclimation groups. Differences in proton leak respiration rates of UCP1-containing cells activated with various concentrations of TTNPB or nonanoic acids were examined using one-way ANOVA. We calculated the UCP1 centre activity of mouse and tenrec UCP1 with a dynamic fitting exponential growth curve (Single, three parameter, f = y 0 + a *exp( b * x )). These analyses were performed using SigmaStat (Jandel Scientific, San Rafael, CA, USA). All mean values were reported±s.e.m., and the 0.05 level of probability was accepted to indicate statistical significance. Accession codes: The sequences generated for this study were deposited in GenBank under accession number KC158558.1 . How to cite this article: Oelkrug, R. et al. Brown fat in a protoendothermic mammal fuels eutherian evolution. Nat. Commun. 4:2140 doi: 10.1038/ncomms3140 (2013).